Global meta-analysis reveals low consistency of biodiversity congruence relationships Knowledge of the number and distribution of species is fundamental to biodiversity conservation efforts, but this information is lacking for the majority of species on earth. Consequently, subsets of taxa are often used as proxies for biodiversity; but this assumes that different taxa display congruent distribution patterns. Here we use a global meta-analysis to show that studies of cross-taxon congruence rarely give consistent results. Instead, species richness congruence is highest at extreme spatial scales and close to the equator, while congruence in species composition is highest at large extents and grain sizes. Studies display highest variance in cross-taxon congruence when conducted in areas with dissimilar areal extents (for species richness) or latitudes (for species composition). These results undermine the assumption that a subset of taxa can be representative of biodiversity. Therefore, researchers whose goal is to prioritize locations or actions for conservation should use data from a range of taxa. Understanding the distribution of biodiversity is central to ecology, and underpins biodiversity conservation efforts such as the prioritization of protected areas [1] , [2] , [3] . Yet information on the number and spatial distribution of species is lacking for the majority of taxa on earth [4] . Although broad-scale patterns of biodiversity are well documented [5] , accurate descriptions of the distribution of biodiversity break down at fine spatial, temporal or taxonomic scales, even for well-described groups such as vascular plants [6] or vertebrates [7] . Further, ongoing efforts to resolve the biases and deficiencies of taxonomic data sets are unlikely to occur quickly enough to allow improved conservation decision making [8] . Therefore, a major goal in ecology is to identify consistent biodiversity patterns that can be used to guide conservation actions despite this considerable uncertainty [9] , [10] , [11] . One solution to the problem of inadequate information on the distribution of biodiversity is to rely on proxies [12] . These proxies are typically metrics describing the richness or diversity of taxonomic or environmental units [13] , which are assumed to be representative of broader patterns of biodiversity. Although this approach avoids the need to detect all species within a given study area, it requires that ecologists assume equivalency among different taxa and that cross-taxon congruence is high; that is, observed taxa are representative of the distribution of unobserved taxa, and therefore of a wider community of co-occurring species. This assumption has critically important implications for biodiversity conservation [13] , [14] , [15] ; where this assumption holds, studies of a single taxon will have broad relevance to other taxa, increasing the value of those studies for addressing the extinction crisis. In contrast, low cross-taxon congruence reduces our ability to identify losses of biodiversity, and therefore our ability to address such losses. Perhaps because of the importance of this issue, a large literature quantifying, discussing and synthesizing knowledge on cross-taxon congruence has emerged. Early work focused primarily on quantifying patterns of species richness [1] , [16] , [17] , [18] , but this approach can fail to adequately represent rare or endemic species [19] , [20] , [21] , thereby limiting its utility for spatial conservation planning [2] , [22] . As a result, recent work commonly supplements or replaces analysis of species richness with methods that account for species identity. This can be achieved either by comparing species composition between taxa using Mantel tests [23] , [24] or by calculating the degree of overlap between optimal subsets of sites for each taxon [25] , [26] (an approach based on the principle of complementarity [27] ). Although these developments have been valuable, they present a challenge to those attempting to synthesize global knowledge on cross-taxon congruence because of the array of different methods that have been applied in the literature [28] , [29] . Therefore, despite the publication of a number of valuable reviews of the congruence literature [15] , [28] , [30] , [31] , [32] , [33] , [34] , one important theme has yet to be addressed; namely, the observation that congruence is often highly variable when measured in different locations or at different times [29] , [35] , [36] . A key property of biodiversity surrogates and indicators is that they should be able to be applied with confidence in novel contexts [37] , and so this lack of consistency has the potential to undermine the usefulness of biodiversity surrogates in ecology and conservation [38] . Although inconsistency in cross-taxon congruence has been clearly demonstrated in a subset of study locations, the extent of the problem, and the identity of factors driving it, remains unclear. However, several variables may have a role in generating dissimilarity in congruence estimates. In particular, biogeographical parameters such as latitude [39] or elevation [40] , [41] influence biotic distributions at global scales, and can therefore influence congruence between taxa as well [42] . Further, considerations of study location and design—such as spatial scale (defined here as the areal extent of the study region), grain size (the size of each sampling unit) or sample size (the number of sampling units in the study)—can strongly influence observed congruence relationships [12] , [13] , [14] , [24] . Finally, different pairs of taxa vary in their degree of congruence [24] , [43] , [44] , but identifying taxon-specific attributes that influence congruence is difficult. One simple approach is to use phylogenetic relatedness as a proxy for ecological traits (such as body size [28] ) that influence congruence patterns. However, this approach can fail at large taxonomic scales [30] owing to low phylogenetic conservatism of species traits [45] or the existence of mutualisms between distantly related taxa [46] . Because of the range of parameters known or suspected to influence biodiversity per se , as well as cross-taxon congruence, we currently lack an overarching view of which parameters most strongly influence both the extent, and the consistency, of cross-taxon congruence across different studies, between locations or through time. To address this key research gap, we ask the question: which attributes of biodiversity studies most strongly influence the extent and consistency of cross-taxon congruence? We address this question using data from a global meta-analysis of the richness, composition and complementarity of terrestrial and freshwater eukaryotic taxa, spanning plants, fungi and 14 animal classes. Further, our analysis includes studies that range in spatial scale from small patches (on the order of ~\n10 km 2 ) to studies encompassing the entire terrestrial surface of the earth. To our knowledge, this is the first attempt to study variables that influence both the extent, and the consistency, of cross-taxon congruence across the ecology and conservation literature. Our meta-analysis shows that variability is the norm for estimates of cross-taxon congruence in the ecology and conservation literature. Although several factors influence the extent of observed cross-taxon congruence, attributes of study design have a much stronger role than bioclimatic or phylogenetic variables in driving congruence relationships. In total, the variables that we investigate explain a low proportion of variance in observed congruence, with 85% of variation remaining unexplained. Our results therefore suggest caution in the application of biodiversity surrogates outside of their initial study locations or times, but also identify new areas of uncertainty and bias in global patterns of cross-taxon congruence, and in the study of biodiversity surrogates more broadly. Broad patterns in the congruence literature Our investigation of the ecology and conservation literature led to the identification of 1,120 reported values of cross-taxon congruence in species richness, composition or complementarity from a total of 74 articles. Most data described congruence in species richness, for which we found 742 usable correlations from 64 articles, with substantially fewer data available for congruence in species composition (274 correlations from 14 articles). Our chosen metric for assessing congruence in complementarity was the Species Accumulation Index (SAI; see ref. 15 ). The SAI is a metric with distinctly different properties from the correlations described elsewhere in this paper. It is calculated by comparing the area under a curve describing the proportion of taxa represented within increasing numbers of sites (O) against similar areas for curves describing the proportion of species incidentally represented from a second (surrogate) taxon (S), and also against randomly ordered sequences of those sites (R) [47] . It is calculated using the formula: Consequently, this metric approaches one as the surrogate and target taxa increase in congruence (that is, where they accrue species at the same rate as the number of sites increases), but can be negative where the surrogate performs worse than randomly selecting sites in terms of representing the target taxon. Further, SAIs differ from correlations in species richness or composition in that their values differ depending on which taxon is the target and which is the surrogate (that is, SAIs give two values for each pair of taxa, in contrast to correlations which give a single value for each pair). We found only six articles (and 104 observations) that used the SAI for assessing the degree of complementarity between taxa, possibly because there are many methods for assessing congruence in the complementarity literature [29] . Although six articles was too few to make broad comparisons regarding the influence of study design or location on observed levels of congruence, we were able to make some broad observations. In particular, when comparing a single pair of taxa, switching the identity of target and surrogate led to a mean difference in observed SAI of 0.20 (56% of the mean). In the most extreme case, switching the identity of surrogate and target taxa led to a change from strongly positive SAI (0.57) to strongly negative (−0.44, a difference of 1.01 comparing accumulation of species from the classes Odonata and Mammalia [26] ). Across all three metrics of cross-taxon congruence that we collected, the vast majority of values were >0 (richness=83%, composition=95% and SAI=91%). Mean congruence in species richness was 0.35, with a s.d. of 0.36; the corresponding value for congruence in species composition was 0.27 (s.d.=0.26), whereas mean SAI had a mean value of 0.36 (s.d.=0.32). These results show that although there is a broad congruence between taxa in general, congruence is not typically high, whereas there is a high degree of variation in congruence between studies. We found evidence of some scale-related biases in our data set. In particular, congruence was rarely studied across the full extent of spatial scales for a given combination of taxa, with few studies of cross-taxon congruence at global scales for orders within the Arthropoda (>10 7 km 2 ), and no studies of species richness congruence between vertebrate classes at fine spatial scales (<100 km 2 ). 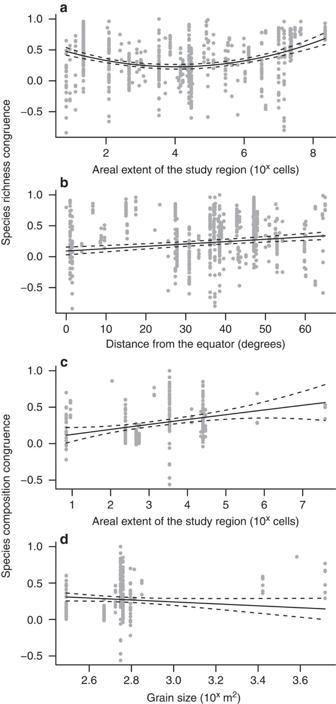Figure 1: Effects of variables that significantly influence congruence in species richness or composition. (a,b) Species richness, and (c,d) species composition. Dashed lines give 95% confidence intervals. Full coefficient estimates and their degree of statistical significance are given inTable 2. There also was bias between metrics in relation to scale, with species compositional congruence being assessed at fine spatial scales when compared with studies of species richness congruence ( Table 1 ). However, this latter point may be a statistical artefact resulting from the paucity of studies using complementarity-based criteria (which tend to replace analysis of species composition at larger spatial scales) in our review, rather than a cause for concern over spatial bias. Table 1 Summary statistics for congruence and spatial scale for commonly studied taxa. Full size table We also observed a clear disconnect between the frequency of taxon use in the literature, and the extent of congruence with the richness or composition of other taxa. Species richness of Coleoptera was the most commonly studied response variable in our data set ( n =198; Table 1 ), but Coleoptera were only the seventh-ranked taxon in terms of average congruence in species richness (mean Pearson’s correlation=0.34). Similarly, Aves was the most common vertebrate taxon in our data set ( n (correlations) =174, 130 of which were for species richness), but displayed the third lowest congruence in species richness (mean Pearson’s correlation=0.29), although Aves did show the highest average congruence in species composition of any taxon (mean Pearson’s correlation=0.40). Further, Coleoptera and Arachnida were the most frequently occurring taxa in our species composition data set ( n (correlations) =64; Table 1 ), but displayed only the fourth and the sixth highest correlations on average (with mean Pearson’s correlations of 0.32 and 0.26, respectively). Extent of cross-taxon congruence Models of congruence showed that spatial scale had the dominant influence on congruence in species richness (metric 1) and composition (metric 2), displaying a significant linear effect on compositional congruence (0.08, s.e.=0.02, P <0.001; Fig. 1c ) and a quadratic influence on species richness congruence (0.12, s.e.=0.02, P <0.001; Fig. 1a ). Grain size had an additional additive effect on congruence in species composition (0.09, s.e.=0.02, P <0.001; Fig. 1d ), but not on congruence in species richness. Latitude significantly influenced congruence in species richness (0.06, s.e.=0.013, P <0.001; Fig. 1b ), but this effect was reduced when the extent of the study region was large (−0.07, s.e.=0.014, P <0.001). 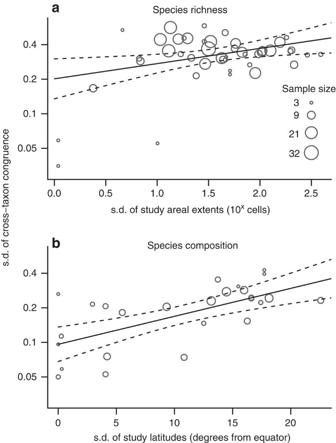Figure 2: Significant predictors of consistency in cross-taxon congruence. Predictors are given for species richness (a) and species composition (b). Points show values for a single pair of taxa, measured across many studies, with the number of studies used to calculate the s.d. (and therefore to weight each point in the linear model) shown by point size. Dashed lines show 95% confidence intervals. Full coefficient estimates and their degree of statistical significance are given inTable 3. Elevation and phylogenetic relatedness had no significant effect on congruence for either metric ( Table 2 ). Despite the identification of several significant predictors for each metric, model fit was poor, with r 2 values of 0.17 and 0.13 for congruence in species richness and composition, respectively. Figure 1: Effects of variables that significantly influence congruence in species richness or composition. ( a , b ) Species richness, and ( c , d ) species composition. Dashed lines give 95% confidence intervals. Full coefficient estimates and their degree of statistical significance are given in Table 2 . Full size image Table 2 Estimated coefficients for all variables in models of cross-taxon congruence. Full size table Our finding of a nonlinear relationship between congruence in species richness and spatial scale highlighted that most studies from our data set focused on scales and metrics where congruence was lowest. In particular, 40% of species richness correlations were measured at areal extents between 1,000 and 100,000 km 2 , that is, at scales where our results showed congruence was generally low. Further, species richness patterns were less congruent at intermediate scales than species composition patterns ( Fig. 1a,c ), but richness correlations were 2.7 times more common in our data set at this scale. Therefore, when working at landscape scales, ecologists should be cautious before assuming that spatial or temporal variation in species richness is representative of variation in total species richness (that is, biodiversity). Consistency of cross-taxon congruence To assess drivers of (in)consistency in cross-taxon congruence, we calculated s.d. values of congruence in species richness for 45 pairs of taxa, with the most commonly studied pair (Coleoptera versus Hymenoptera) having a total of 32 observations (mean n (correlations) =9.5). We found a significant effect of spatial scale on inter-study variation in species richness congruence (0.21, s.e.=0.08, P =0.01; Fig. 2a ), but no evidence of an effect of variation in grain size, latitude or elevation ( Table 3 ). Data on congruence in species composition were more sparse, with only 26 pairs of taxa represented in this data set (mean n (correlations) =5.3). Inter-study variation in congruence of species composition was significantly higher where studies occurred across a range of latitudes after weighting by sample size (0.51, s.e.=0.11, P <0.001; Fig. 2b ), but there was no significant effect of spatial scale. Figure 2: Significant predictors of consistency in cross-taxon congruence. Predictors are given for species richness ( a ) and species composition ( b ). Points show values for a single pair of taxa, measured across many studies, with the number of studies used to calculate the s.d. (and therefore to weight each point in the linear model) shown by point size. Dashed lines show 95% confidence intervals. Full coefficient estimates and their degree of statistical significance are given in Table 3 . Full size image Table 3 Effect of variance in study design and location parameters on inter-study variance in congruence. Full size table We completed an extensive meta-analysis of the extent of cross-taxon congruence from a range of studies covering an ambitious spatial and taxonomic scope. Our analysis revealed that high variance in cross-taxon congruence is the norm in the ecology and conservation literature. This suggests that there are few circumstances in which pairs of taxa will be consistent surrogates for each other across a range of metrics, locations and spatial scales [35] , despite most studies returning estimates of cross-taxon congruence that are >0. Further, variables describing the spatial scale of congruence studies, as well as biogeographic and phylogenetic parameters, explain limited variance in cross-taxon congruence, even though they are well-known proxies for broad-scale and globally important biological processes [39] , [40] . Our results therefore highlight several important sources of bias and uncertainty in the literature on biodiversity surrogates. Although the influence of spatial and biogeographic parameters on cross-taxon congruence was limited, it is clear that the spatial scale of a study—and, to a lesser extent, its latitude—has a role in determining the extent of congruence observed in that investigation [34] . This important result extends an array of earlier work, showing that the scale at which studies are conducted can influence study outcomes, such as the distribution of biodiversity hot spots [7] , [12] , or the relationship between species distributions and underlying environmental parameters [48] , [49] . It also suggests a need for caution when synthesizing research on processes that vary across spatial scales. For instance, Mellin et al. [31] report linearly decreasing congruence with increasing spatial scale in marine environments, whereas others have reported results entirely opposite to ours (namely, lowest congruence at extremes of spatial scale) [8] , [30] . However, these differences are clearly attributable to methodological considerations: Mellin et al. [31] use >100 km 2 as their highest category of spatial extent, six orders of magnitude lower than our maximum recorded values, whereas Wolters et al. [30] use analysis of grain size rather than spatial extent. These are independent metrics that—as we and others have shown—have differing effects on observed patterns of biodiversity [35] , [50] . These contrasts show that the choice of scales—and the metrics used in assessments of the effects of scale—can strongly influence the outcome of ecological studies and meta-analyses, and can thereby influence inferred patterns of biodiversity [35] , [50] . We found no evidence for an effect of higher-level phylogeny on cross-taxon congruence, a result that has several key implications. First, it suggests that the long-discussed bias towards vertebrates in the ecology literature [51] , [52] might be less of a problem than previously thought, because our results give no a priori reason to anticipate that vertebrate and invertebrate distributions will be incongruent [17] , [53] (although some clearly are [54] ). Second, our finding of no relationship between congruence and relatedness as this level of taxonomic aggregation (that is, at the Order level or above) also causes problems for researchers aiming to quantify the distribution of biodiversity in general [45] ; any results will probably apply to some other taxa, but we have no way of knowing which ones. Therefore, future work should aim to investigate precisely which taxa are consistent surrogates for each other, and what processes drive these surrogacy relationships (see below). Our study also revealed significant bias in the literature, such that there were few studies of vertebrates at fine spatial scales (<10 4 km 2 ) and few global-scale studies (>10 6 km 2 ) of congruence in arthropods. However, these trends are likely to be the result of methodological difficulties. For example, many vertebrates routinely move distances ranging from metres to kilometres to forage, making it unclear whether assessing the ‘distribution’ of vertebrates at finer spatial scales than these routine movements is particularly meaningful [55] . Conversely, taxonomic completeness is low for many arthropod taxa as a result of their enormous diversity [56] , perhaps accounting for their lower use in global-scale biodiversity assessments. Fortunately, this appears to be changing, with some recent studies greatly expanding the scale at which patterns of invertebrate biodiversity are investigated (see, for example, ref. 53 ). The pattern that we have observed in the ecology literature of variable and context-dependent congruence, combined with bias towards a narrow subset of taxonomic groups, has important conservation implications. In particular, we found that congruence in species composition was low below 10 3 km 2 ( Fig. 1c ), suggesting that at these fine spatial scales complementarity-based metrics applied to single taxa are unlikely to be broadly representative of biodiversity [50] . In contrast, species richness is a metric that is most commonly applied at landscape scales (~\n10 3 km 2 ), that is, at precisely those scales where observed patterns will be least well correlated with overall biodiversity [50] , [57] . This implies that ecologists that monitor change in species richness over time (for example, as an indicator of ecological change) at landscape scales should strongly consider monitoring a number of functionally distinct taxonomic groups if their recommendations to managers are to be robust. Our results question the generalizability of biodiversity surrogate relationships (see also refs 29 , 58 ), but we do not suggest that surrogates are without value. Instead, we suggest that there is considerable scope for a shift in emphasis away from repeating research on taxa that display low average congruence. Instead, future research should focus on consistency as an indicator of the usefulness of potential biodiversity surrogates. Given the low consistency that we have described above, however, new approaches to studying cross-taxon congruence may be required. For example, one option may involve identifying sets of taxa that—when used in combination—may act as surrogates for a broader subset of biodiversity than each would alone. Identifying sets of taxa with these properties might be aided by systematic testing of rarely studied taxa (or rarely studied combinations of taxa) as biodiversity surrogates [53] . Regardless of the adoption of these suggestions, however, a useful first step would be for researchers to articulate their reasons for anticipating that a given taxon will be a consistent surrogate for other taxa [59] , rather than choosing surrogates on the basis of prior experience with that taxon. Further work also is required to identify the extent to which species-, genus- or family-level traits influence cross-taxon congruence [28] . Clearly, there are limits to the practice of using relatedness among higher clades as a proxy for shared traits [60] , [61] , particularly as environmental gradients can cause high congruence of taxa with very different phylogenetic histories [62] , [63] . One useful question to answer, therefore, would be whether relatedness has a useful level of explanatory power when used to investigate congruence between more closely related taxa than we have investigated here (that is, at the family level or below) [11] , [64] ; or conversely, whether there are situations where the collection of further taxonomic or phylogenetic information is unhelpful and should be abandoned in favour of environmental or habitat-based biodiversity surrogates [65] , [66] , [67] . Comparisons of the usefulness of functional and phylogenetic metrics of diversity [68] also should be considered as potential means to improve surrogacy and conservation decisions. In this paper, we addressed a question of key importance for advancing the understanding and application of biodiversity surrogates by investigating patterns and drivers of consistency in biodiversity congruence. Using a meta-analysis approach, we have shown that estimates of cross-taxon congruence vary enormously, even for the same pairs of taxa, and after the influence of spatial and biogeographic parameters are taken into account. Further, we also demonstrated that congruence relationships are not predictable from information on relatedness at the Order level (or above), thereby limiting our understanding of the generality of such relationships. The clear implication of these findings is that cross-taxon congruence cannot be assumed. Consequently, research on the distribution of biodiversity will be misleading where researchers rely on data from a single taxon; a result with clear but troubling implications for the effectiveness of management interventions informed by that research. Future work should clearly elucidate—and, if possible, test–the range of locations, scales or taxa over which any observed congruence relationships are expected to apply. Conceptual scope We defined cross-taxon congruence as congruence that was calculated for two non-overlapping clades. This definition placed three important restrictions on the kind of studies that we were able to consider in our meta-analysis. First, we considered only studies of cross-taxon congruence and not the other forms of congruence that occur regularly in the biodiversity surrogate literature [31] . Within-taxon congruence occurs where species-level diversity of a subclade is taken as representative of species-level diversity of the whole taxon, whereas higher-taxon congruence occurs where species-level diversity is tested against the diversity of genera, families or orders in the same broad taxonomic group. In both cases, it is difficult to define the degree of phylogenetic relatedness between target and surrogate taxa. Consequently, only cross-taxon surrogates allow us to investigate whether closely related taxa are more highly congruent on average than distantly related taxa, and so we excluded studies of within-taxon or higher-taxon congruence from our analysis. Second, we considered only studies that investigated congruence in species richness, composition or the SAI. This excludes endemism because it is typically quantified at continental or global scales [2] , which means that we could not evaluate how endemism varies with scale. In contrast, we restricted our assessment of complementarity metrics to the SAI following the reasoning given by Rodrigues and Brooks [15] . Third, we used only taxonomically defined groups in our analysis. This led to exclusion of several categories of surrogates as follows: (1) functionally similar but poly- or paraphyletic groups such as epiphytes, lianas or herpetofauna; (2) mutualists such as lichens; (3) structural attributes of vegetation; and (4) subsets of taxa defined by functional traits such as body size (for example, small mammals) or behaviour (for example, breeding birds). Article identification We used a multi-stage approach to identify relevant articles. In particular, we required a straightforward approach for evaluating the very large literature on surrogates in ecology, and so we automated a number of stages using the R language environment [69] . Our first stage involved running a search for articles using both Scopus and ISI ‘web of knowledge’ databases. We ran our ISI search on the 22 November 2012, and requested all articles mentioning either of the terms ‘surrogate’ or ‘indicator’ in their topic from the field of environmental sciences and ecology. We further restricted our search to the following research areas: marine and freshwater biology, biodiversity conservation, fisheries, zoology, remote sensing, plant sciences, mycology, evolutionary biology or forestry. We ran our Scopus search using the same search terms on the 8 January 2013. Our ISI search gave 11,004 articles, whereas our Scopus search gave 36,718 articles for a combined total of 47,722 articles (before removal of duplicates). Our second stage was to identify taxonomic groups that were discussed in each article. We achieved this by searching for taxonomic names in article titles or abstracts using the findIT tool provided by the uBio project ( http://www.ubio.org ). This approach automatically recognizes taxonomic identifiers in strings of text. From these results, we then created a database of unique taxonomic identifiers and re-queried the database to acquire higher-level taxonomic information on each taxon. We also identified a set of common names associated with these taxonomic identifiers and re-searched all article titles and abstracts to find taxa listed only by common names. After manually checking both databases to avoid errors, we were left with 5,943 scientific names and 1,081 common names. Only 7,997 articles (17%) contained at least one taxonomic identifier, suggesting either that our search terms included a number of irrelevant articles or that few articles described their study taxon in the title or abstract. Our third stage was to determine which articles discussed multiple taxonomic groups. We created taxonomic groups of interest by identifying articles that mentioned eukaryote versus prokaryote taxa. Where a taxonomic classification at that level of the taxonomic hierarchy contained more than 1,000 articles, we split that article into the next lowest level in the taxonomic hierarchy. We continued this process until splitting resulted in groups that were too small for meaningful analysis (typically the Class level, although we split insects into Orders). We then identified all articles that mentioned three or more distinct taxonomic groups ( n =689) and used this subset for subsequent analysis stages. Our fourth stage was to identify articles that quantified cross-taxon congruence. We achieved this by reading the abstracts of the remaining 689 articles and marking those that were likely candidates to contain information on the correlation in species richness or composition between pairwise combinations of taxa. We found 76 articles that were likely candidates, but upon searching the full articles only 32 contained usable data. Because our automated approach had the potential to exclude relevant articles, we then searched the reference lists of the 76 most relevant articles to identify any further articles of interest. This gave a further 389 articles, of which 49 were newly identified articles containing data. This left us with a total of 81 articles containing data appropriate to our questions about cross-taxon congruence. We added information on complementarity to our analysis using a supplementary search on 23 January 2014. We searched for all articles matching an ISI search ‘complementarity and surrogates’ from either of the fields of ‘environmental sciences and ecology’ or ‘biodiversity conservation’. We then added any articles that were cited by Rodriguez and Brooks [15] , or had cited either that article or Williams et al. [22] , giving us a total of 220 new articles. We also added articles that had earlier been excluded from our analysis for containing only complementarity-based criteria ( n =39), and all of the articles that we had downloaded to this point ( n ~\n200 articles). Finally, we read all of these articles to identify examples where the authors had used SAI to compare congruence between two taxa. This left us with six articles for inclusion in our analysis. Extraction of correlations For all articles, we looked for cross-taxon congruence in species richness, composition or complementarity. Where data were unavailable, listed only P values or provided only correlations for statistically significant values, we contacted the authors for the raw correlations. Where this information was not available, we excluded that article from further analysis to avoid publication bias. Where an author provided raw data but not correlations, we calculated (Pearson’s) correlations ourselves. We used species richness data that were generated in a number of ways as follows: raw counts of species richness; extrapolated richness calculated using rarefaction; area-adjusted richness calculated by regression or species area curves; species density; or gradient-adjusted richness (that is, after removal of dominant trends besides area). We also used data from studies of any design, including those that used field-recorded observation data; atlas data sets or counts of museum records within grid cells; or studies that estimated broad-scale richness patterns using overlaid range maps. Correlations in species richness were included regardless of whether they were calculated using Spearman’s, Pearson’s or Kendall’s correlations. If there was a choice, we used correlations based on raw data rather than transformed data. The data on species composition that we identified during our review were much more diverse than species richness data. We included only methods that calculated a distance metric between sites and performed some form of correlation on those distance matrices (such as Mantel tests). However, we retained studies that used either abundance or occurrence data, and therefore our data set includes studies that used a range of transformations and distance calculations. Where a study gave separate results for congruence derived from both abundance and occurrence matrices, we used abundance only to avoid pseudo-replication. Although the differences between different composition evaluation methods are important, we did not anticipate that they would make a difference in the direction of congruence relationships. We anticipated, however, that our composition data would have comparably higher noise than our species richness data as a result of methodological inconsistencies between studies. In addition to our response variables, we calculated several predictor variables, using information from a range of sources. We calculated spatial scale as the number of 30 arc-second pixels within a rectangular region defining the study region. Where details of the study region were not given, we took the maximum and minimum latitude and longitude, and calculated the study region as the rectangle bounded by these values. Study latitude was defined as the central point of this study region, measured as distance from the equator in decimal degrees (that is, all latitudes were positive definite). Similarly, our mean elevation results were calculated for these same regions, using freely available digital elevation data from http://www.worldclim.org , which we analysed using the ‘raster’ package [70] in the R statistical programme [69] . Finally, we used the ‘TimeTree’ online data set ( http://timetree.org ) to determine the mean relatedness between pairwise combinations of taxa. TimeTree gives an estimated number of million years since the common ancestor for any combination of taxa that are in its repository. Consequently, this metric is particularly useful for analyses of broad differences between dissimilar taxa, such as we use in this paper. Statistical methods We tested the effect of study-related covariates on the extent of cross-taxon congruence by first splitting our data set into correlations of species richness and species composition, and then constructing a single linear model for each of these two response variables. Predictor variables included in each model were areal extent (measured by log10 ½ degree cells), areal extent squared (as before, but included to test for curvilinear relationships between scale and congruence), grain size (log10 m 2 ), latitude (degrees from equator), elevation (metres) and phylogenetic distance (log10 million years since common ancestor). The only difference between models for species richness and composition was that our species richness model included global-scale studies, for which latitude values (zero) were potentially misleading; hence this model included an interaction between latitude and areal extent that was missing from the species composition model. We assessed consistency of cross-taxon congruence by identifying all pairwise comparisons of our taxa that occurred in each data set on three or more occasions. We then calculated the s.d. of observed congruence across all the studies for each pair. This left us with a data set in which each observation gave the s.d. of observed correlations for that taxon. We then created four linear models, in which the s.d. of correlations was the response variable, and one of the s.d. values of scale, grain size, latitude and elevation were predictor variables. In each model ( n =8), the influence of each pair of taxa to the regression was weighted by the natural log of the number of correlations used to calculate the s.d. (that is, sample size) to account for the fact that low sample sizes can lead to misleading estimates of the s.d. We ran all of our analyses in the R statistical programme [69] , and assessed the statistical significance of variables in each of our models using the t -statistic. How to cite this article: Westgate, M. J. et al. Global meta-analysis reveals low consistency of biodiversity congruence relationships. Nat. Commun. 5:3899 doi: 10.1038/ncomms4899 (2014).